Engineering RNA endonucleases with customized sequence specificities Specific cleavage of RNAs is critical for in vitro manipulation of RNA and for in vivo gene silencing. Here we engineer artificial site-specific RNA endonucleases to function analogously to DNA restriction enzymes. We combine a general RNA cleavage domain with a series of Pumilio/fem-3-binding factor domains that specifically recognize different 8-nucleotide RNA sequences. The resulting artificial site-specific RNA endonucleases specifically recognize RNA substrates and efficiently cleave near their binding sites. The artificial site-specific RNA endonucleases can be devised to recognize and cleave various RNA target sequences, providing a useful tool to manipulate RNAs in vitro . In addition, we generate designer artificial site-specific RNA endonucleases to specifically silence an endogenous gene in Escherichia coli , as well as a mitochondrial-encoded gene in human cells, suggesting that artificial site-specific RNA endonucleases can serve as a gene-silencing tool with designed specificity. The discovery of type II DNA restriction enzymes nearly 40 years ago marked the birth of the recombinant DNA era. However, despite extensive investigations, an equivalent enzyme that cleaves RNA in a sequence-specific manner has not been found in nature. The known RNA endonucleases either cleave their targets through recognition of specific structures (for example, RNase III family or RNase H) [1] , [2] or have limited sequence specificity (for example, RNase A or RNase T1). The molecular machineries that mother nature has evolved for sequence-specific RNA cleavage (for example, RNA interference (RNAi) machinery) involve multi-component complexes that require a guide RNA for target recognition and a protein–RNA assembly for activity, limiting their application in probing structured RNA or manipulating recombinant RNA in vitro . As a gene-silencing method, RNAi is also restricted to target mRNA in the organisms with a reliable RNAi pathway, thus it cannot cleave RNA in other cellular compartments (such as mitochondrial RNA) or be used in some parasitic protozoa (such as Leishmania and Plasmodium ) [3] . Previously, the hammerhead ribozymes, or DNAzymes and PNAzymes, have been engineered to achieve site-specific RNA cleavage [4] , [5] . However, these nucleic acid enzymes generally have low turnover rates compared with protein enzymes, possibly due to tight binding to their substrates. The application of such nucleic acid enzymes is further compromised by the high production cost and low stability of RNA, as well as by the lack of control over folding of single-stranded RNA or DNA. Therefore, it is highly desirable to create RNA 'restriction enzymes' as simple proteins that can be produced with general recombinant protein technologies and expressed in various cells with different gene expression systems. We have engineered a new class of endoribonucleases, called artificial site-specific RNA endonucleases (ASREs), which can specifically recognize an 8-nucleotide (nt) RNA sequence and make a single cleavage in the target. We further determined the cleavage sites and the kinetics parameters of these new enzymes. Our data indicate that these endoribonucleases are capable of efficiently and specifically cleaving diverse RNA targets not only in vitro , but also in cultured cells. To our knowledge, this work marks the first reported restriction enzyme for RNA, which may have important implications in the development of new RNA-engineering technologies and gene-silencing methods. Design of ASREs To create a 'restriction enzyme' for RNA, we adopted a modular design by combining a target recognition domain and a catalytic domain. For the target recognition domain, we chose the unique RNA binding domain (Pumilio/fem-3-binding factor (PUF) domain) of human PUM1 that contains eight repeats to recognize eight consecutive RNA bases [6] , [7] ( Fig. 1a ). Two amino acids in each repeat specifically interact with the Watson–Crick edge of each corresponding base. Thus, by modifying these amino acids in each repeat, a PUF domain can be reprogrammed to bind any 8-nt RNAs [6] , [7] , [8] , [9] . For the RNA cleavage module, we used the PIN domain (PilT amino terminus) of SMG6, which is a non-specific endonuclease domain with well-defined molecular architecture and requires only a divalent cation for its activity [10] , [11] , [12] ( Fig. 1a ). We connected the two domains with a heptapeptide linker (VDTGNGS) designed based on the amino acid propensity of natural linkers in multi-domain proteins [13] . The detailed procedures for ASRE construction were shown in Supplementary Methods and Supplementary Table S1 . 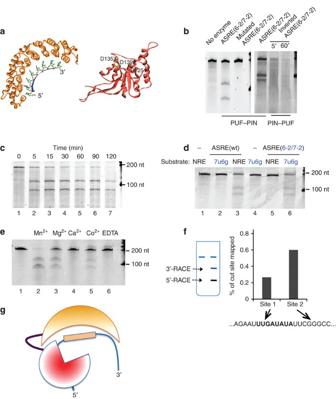Figure 1: Design and biochemical characterization of ASREs. (a) Structures of the PUF domain of human pumilio1 (PDB ID: 1M8W) bound by NRE-19 RNA target (left) and the PIN domain of Smg6 (right; PDB ID: 2HWW). Three Asp residues (indicated in green) near PIN-active site were marked. (b) ASRE with PUF–PIN configuration was incubated with a cognate RNA substrate for 30 min, and the products were resolved in urea–PAGE gel. Inverted ASRE (PIN–PUF) was also tested with the same reaction condition (lane 5 and 6). (c) Time course of RNA digestion by ASRE(6-2/7-2). Digestion was followed in the standard reaction buffer containing 3 mM Mn2+. (d) RNA substrates containing either an NRE site (5′-UGUAUAUA-3′) or 7u6g site (5′-UugAUAUA-3′) were incubated with ASRE(wt) or ASRE(6-2/7-2). The cognate target–ASRE pairs were indicated with same colour. Lanes 1 and 4 are controls without enzyme. (e) The RNA cleavage activities of ASREs are dependent on different divalent metal ions. In all lanes, the concentrations of metal ions were 3 mM. (f) ASRE cleavage site was mapped by 5′- and 3′-RACE using gel-purified RNA products. The positions of two cleavage sites are indicated with arrows and the relative frequencies are plotted. The 8-nt binding sequence of PUF is shown in bold. (g) The 'curve back' model of ASRE best explains the cleavage positions mapped inf. Figure 1: Design and biochemical characterization of ASREs. ( a ) Structures of the PUF domain of human pumilio1 (PDB ID: 1M8W) bound by NRE-19 RNA target (left) and the PIN domain of Smg6 (right; PDB ID: 2HWW). Three Asp residues (indicated in green) near PIN-active site were marked. ( b ) ASRE with PUF–PIN configuration was incubated with a cognate RNA substrate for 30 min, and the products were resolved in urea–PAGE gel. Inverted ASRE (PIN–PUF) was also tested with the same reaction condition (lane 5 and 6). ( c ) Time course of RNA digestion by ASRE(6-2/7-2). Digestion was followed in the standard reaction buffer containing 3 mM Mn 2+ . ( d ) RNA substrates containing either an NRE site (5′-UGUAUAUA-3′) or 7u6g site (5′-UugAUAUA-3′) were incubated with ASRE(wt) or ASRE(6-2/7-2). The cognate target–ASRE pairs were indicated with same colour. Lanes 1 and 4 are controls without enzyme. ( e ) The RNA cleavage activities of ASREs are dependent on different divalent metal ions. In all lanes, the concentrations of metal ions were 3 mM. ( f ) ASRE cleavage site was mapped by 5′- and 3′-RACE using gel-purified RNA products. The positions of two cleavage sites are indicated with arrows and the relative frequencies are plotted. The 8-nt binding sequence of PUF is shown in bold. ( g ) The 'curve back' model of ASRE best explains the cleavage positions mapped in f . Full size image We first constructed an ASRE in the PUF–PIN configuration from N- to carboxy terminus using a modified PUF(6-2/7-2) that specifically binds 5′-UugAUAUA-3′ (7u6g, see Methods and Supplementary Table S2 ) [7] . The recombinant ASREs were purified ( Supplementary Fig. S1 ) and incubated with a 191-nt RNA substrate containing its cognate 8-nt target. We observed a rapid cleavage of the substrate into two fragments with expected sizes. In contrast, the control ASRE with an inactive PIN domain (D1353A mutation in PIN-active site [11] ) had no detectable activity ( Fig. 1b ), suggesting that the cleavage was indeed catalysed by the PIN domain. The RNA cleavage was nearly complete within 2 h ( Fig. 1c ). An inverted ASRE with PIN–PUF configuration showed non-specific RNA cleavage ( Fig 1b ); we thus chose the PUF–PIN orientation in our subsequent studies. Sequence specificity and ion requirement of ASREs To test for specificity, we created an ASRE containing the wild-type (wt) PUF that recognizes the nanos response element (NRE: 5′-UGUAUAUA-3′) that differs from the PUF(6-2/7-2) target by two nucleotides [7] . The ASRE(wt) cleaved only the substrate containing the NRE sequence ( Fig. 1d , lane 3) but not the closely related 7u6g sequence (lane 2). Conversely, the ASRE(6-2/7-2) specifically cleaved its cognate target but not the NRE-containing substrate ( Fig. 1d ). In addition, the ASRE(6-2/7-2) failed to cleave other closely related RNAs that vary by three to five nucleotides from its substrate ( Supplementary Fig. S2 and Supplementary Table S2 ), suggesting that the ASRE activity is highly sequence-specific. Consistent with the metal-ion selectivity of the PIN domain [11] , we detected optimal activity of ASRE in the presence of Mn 2+ and suboptimal activity in the presence of Mg 2+ ( Fig. 1e ). We made a new observation that the PIN domain may use Co 2+ as a low-activity substitute, as weak ASRE activity was observed in the presence of Co 2+ ( Fig. 1e , lane 5). Although single-stranded DNA can inhibit the non-specific nuclease activity of PIN [11] , it did not affect the specific cleavage by ARSE ( Supplementary Fig. S3 ). This is consistent with the fact that PUF domains do not bind single-stranded DNA [6] . We further measured the initial cleavage rates ( Supplementary Fig. S4a ) to estimate the kinetic parameters of four related ASREs ( Supplementary Table S3 ). The ASRE-catalysed RNA cleavage roughly followed a Michaelis–Menten-like kinetics in our assay conditions ( Supplementary Fig. S4 ), and the cleavage was fairly efficient with k cat /K M around the 10 7 M −1 min −1 range and K M around the 1–3 μM range. This is an approximate estimation as the ASRE proteins were assumed 100% active in the calculations and the initial rates were measured in a 5-min reaction due to our detection limit. In the future, a more detailed enzyme kinetics study will facilitate the optimization of ASREs. Determining cleavage site of ASREs Our data indicated that ASRE-mediated RNA cleavage occurs near the cognate binding site, generating two products whose combined length roughly equals to the length of input RNA as judged by urea–polyacrylamide gel (PAGE). To determine the exact site of ASRE cleavage, we cloned and sequenced both the 5′- and 3′-digestion products from the same reaction using 5′- and 3′-RACE ( Supplementary Fig. S5a,b ). Because of a polyadenylated fragment added during cloning processes, the resulting products do not form a band with a fixed size ( Supplementary Fig. S5c ). We sequenced 41 clones in total to determine the 5′- and 3′-sites, and analysed cleavage sites supported by multiple clones. The fact that digested products can be cloned with RACE indicated that RNA cleavage catalysed by ASRE generates a 5′-fragment with 3′-hydroxyl group. Two cleavage sites (site 1 and 2) were identified by 5′- and 3′-RACE ( Fig. 1f ). The cleavage products of the major site were matched to the same position using both 5′- and 3′-RACE ( Supplementary Fig. S5c ), suggesting the ASRE makes a single cut in each RNA molecule. The major site was located 4 bases downstream of the PUF-binding site and accounted for ~60% of sequenced clones, whereas the minor site was in the third position of the 8-nt PUF-binding site ( Fig. 1f ). As PUF binds RNA in an anti-parallel fashion with the first repeat at the N terminus recognizing the eighth RNA position, such a cleavage pattern indicated that ASREs probably forms a 'fold-back' structure with the RNA substrate being bound by the one arm (PUF domain) and the catalytic PIN domain folding back to cleave the phosphodiester backbone at downstream sites ( Fig. 1g ). We also observed minor cleavage sites near the PUF-binding sequence that were mapped by single clones; such sites could be accounted for by experimental artefact of RNA amplification with RACE, by incomplete ASRE digestion, or by flexibility of the ASRE–RNA complex. In addition, the fact that RNA can also form secondary and tertiary structure in solution adds complexity to this model. The exact mechanism as to how ASREs select the cleavage sites will require determining the three-dimensional structure of an ASRE–RNA complex. Length and structure of linker affects ASRE activity We further examined how different linkers affected the activities of an ASRE. A suitable linker is key to high catalytic activity; however, designing the linker is a major challenge because of lack of prior knowledge of domain flexibility imparted by inter-domain structures. A linker longer than what is necessary to connect two domains may be too flexible and thus could act as an energetic, structural, or activity-interfering nuisance [14] . On the other hand, a short linker may generate a structural barrier that prevents simultaneous contact of the two domains with the RNA substrate. A database of known linkers revealed that both short (< 6 amino acids) and long linkers (>14 amino acids) are very rare in nature, and a typical linker is 6–12 amino acids in length mostly in helical structures [13] . To optimize the ASRE linker length, we designed tripeptide (VDT; 7.3 Å), heptapeptide (VDTGNGS; 12 Å) and dodecapeptide (VDRRMARDGLVH; 20.5 Å) linkers, and inserted them between PUF(6-2/7-2) and wt PIN ( Fig. 2a ). These peptides have mixed helical propensity and should provide limited flexibility to prevent non-native interactions between domains ( http://www.ibi.vu.nl/programs/linkerdbwww/ ). 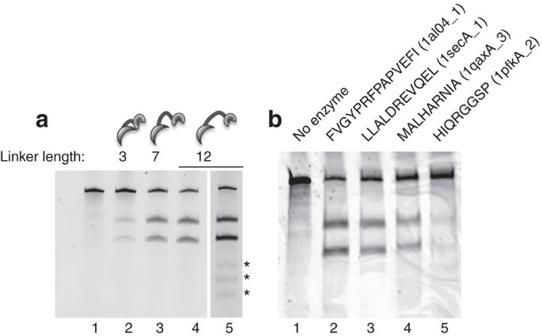Figure 2: Effects of linker length and structure on ASRE activity. (a) The linker length affects the ASRE activity. In lanes 1–4, all reactions were stopped after 30 min incubation. At longer reaction time (60 min), non-specific digestion products (indicated by asterisks in lane 5) were observed with ASRE containing a dodecapeptide linker. (b) The ASRE(6-2/7-2) containing different linker sequences were incubated with its cognate substrate and the cleavage of the RNA was detected with urea–PAGE gel. The different linkers were chosen from the protein inter-domain linker database. Both the sequence and the PDB code were shown. The secondary structures of the linkers are: 1al04_1: HHHHTTCCCCCCCHHHH; 1sesA_1: HHHHHHHHHHH; 1qaxA_3: HHHHTTTHHH; 1pfkA_2: CGGGGGCSCC. The notation of secondary structure follows the standard DSSP code (H, α-helix; T, hydrogen-bonded turn; C, coil; G, 310helix; S, bend). The structures of inter-domain linkers were determined in the natural context of respective proteins. Two amino acids (VD, contributed by theSalI site) were preceded in each peptide. Figure 2: Effects of linker length and structure on ASRE activity. ( a ) The linker length affects the ASRE activity. In lanes 1–4, all reactions were stopped after 30 min incubation. At longer reaction time (60 min), non-specific digestion products (indicated by asterisks in lane 5) were observed with ASRE containing a dodecapeptide linker. ( b ) The ASRE(6-2/7-2) containing different linker sequences were incubated with its cognate substrate and the cleavage of the RNA was detected with urea–PAGE gel. The different linkers were chosen from the protein inter-domain linker database. Both the sequence and the PDB code were shown. The secondary structures of the linkers are: 1al04_1: HHHHTTCCCCCCCHHHH; 1sesA_1: HHHHHHHHHHH; 1qaxA_3: HHHHTTTHHH; 1pfkA_2: CGGGGGCSCC. The notation of secondary structure follows the standard DSSP code (H, α-helix; T, hydrogen-bonded turn; C, coil; G, 3 10 helix; S, bend). The structures of inter-domain linkers were determined in the natural context of respective proteins. Two amino acids (VD, contributed by the Sal I site) were preceded in each peptide. Full size image We found that the purified ASRE with a tripeptide linker had very low activity compared with the other two enzymes ( Fig. 2a , lane 2). The enzymes had considerably higher activities with linker lengths of 7 or 12 amino acids. However, non-specific cleavage products became apparent at longer incubation time with the 12 amino acid linker ( Fig. 2a , lane 5), probably because of excessive flexibility that allowed the PIN endonuclease domain to access and cleave non-cognate sites. Furthermore, the secondary structure of peptide linkers may also affect the efficiency of ASRE-mediated RNA cleavage. When assuming that the inter-domain linker in ASRE would adopt a structure similar to that in their native contexts, we found linkers with α-helical or helix-coil-helix structures produced more active ASREs, whereas linkers with 3 10 helix structures reduced the activity ( Fig. 2b ). Silencing gene expression with ASRE in living cells A potential application of this new class of enzymes is to customize ASREs that specifically silence gene expression, which is especially useful in places where the RNAi machinery is not present. As a proof of concept, we designed an ASRE to target the lacZ transcript in Escherichia coli . We engineered the ASRE(LacZ) by changing PUF repeats 2, 3 and 6 to specifically recognize 5′-UggAUgaA-3′ sequence in positions 1232–1239 and 1520–1527 of the lacZ . We used BL21(DE3) cells in which expression of the ASRE and lacZ can be induced by isopropyl-β- D -thiogalactoside (IPTG). The controls include the non-specific ASRE(87621) that targets a different sequence and the mutated ASRE(LacZ) containing a D1353A mutation in the PIN-active site. We found that the bacteria expressing ASRE(LacZ) had significantly decreased β-galactosidase activity compared with empty vector controls or non-specific ASRE controls ( Fig. 3a ). Consistent with in vitro results ( Fig. 1b ), the ASRE(LacZ) with an inactive PIN domain have essentially no effect, suggesting that the decrease is due to mRNA cleavage by ASRE(LacZ) rather than a translational inhibition. We further measured the steady-state RNA level of the lacZ transcript and found that expression of ASRE(LacZ) significantly decreased lacZ RNA compared with the empty vector or control ASRE ( Fig. 3b ). ASRE(LacZ) with a D1353A mutation in the PIN domain had some residual activity and decreased the LacZ RNA level by half, consistent with reports that this mutation cannot completely eliminate PIN activity in vivo [10] , [11] . The β-galactosidase protein levels were also decreased by ASRE(LacZ) as judged by western blots ( Supplementary Fig. S6 ). This effect is not due to differential expression of ASREs, as the ASRE levels in all clones were roughly equal ( Supplementary Fig. S6 , bottom panel). As a control, expression of the PIN domain alone caused non-specific degradation of total RNA ( Supplementary Fig. S7 ), generating a smear of short RNA fragments in the urea–PAGE gel. This is consistent with previous reports that the PIN domain functions as a non-specific RNA endonuclease [10] , [11] . As expression of the PIN domain is toxic to E. coli cells, a complete degradation of total RNA was not observed ( Supplementary Fig. S7 ). 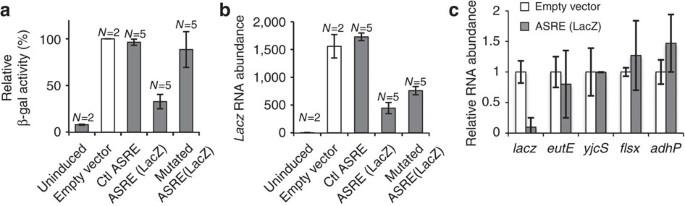Figure 3: Using ASRE to silence gene expression inE. coli. (a) The activity of β-galactosidase (β-gal) inE. colistrains transformed with ASRE(LacZ) plasmid and control plasmids. For each strain, the β-gal activity from multiple independent clones (N=2 or 5) in triplicate experiments was measured. The relative β-gal activity was normalized to clones transformed with the empty vector and induced with the same condition. The uninduced clones containing empty vector was used as the baseline activity. Error bars represent the s.e. across all clones. (b) The levels oflacZmRNA were measured by quantitative RT–PCR. The samples were in the same order as panela.LacZlevels were normalized toftsZmRNA, and the relative RNA abundances compared with uninduced controls are plotted. Error bars represent the s.e. across all clones. (c) The effect of ASREs on other mRNAs containing similar recognition sites. TheE. colistrains transformed with ASRE(LacZ) or empty vector were induced with IPTG, and the RNA levels were measured with quantitative RT–PCR. The relative RNA abundances compared with vector controls are plotted. Two independent clones were selected in each strain, and the inductions were carried out in triplicates. Error bars represent the standard derivations. Figure 3: Using ASRE to silence gene expression in E. coli . ( a ) The activity of β-galactosidase (β-gal) in E. coli strains transformed with ASRE(LacZ) plasmid and control plasmids. For each strain, the β-gal activity from multiple independent clones ( N =2 or 5) in triplicate experiments was measured. The relative β-gal activity was normalized to clones transformed with the empty vector and induced with the same condition. The uninduced clones containing empty vector was used as the baseline activity. Error bars represent the s.e. across all clones. ( b ) The levels of lacZ mRNA were measured by quantitative RT–PCR. The samples were in the same order as panel a . LacZ levels were normalized to ftsZ mRNA, and the relative RNA abundances compared with uninduced controls are plotted. Error bars represent the s.e. across all clones. ( c ) The effect of ASREs on other mRNAs containing similar recognition sites. The E. coli strains transformed with ASRE(LacZ) or empty vector were induced with IPTG, and the RNA levels were measured with quantitative RT–PCR. The relative RNA abundances compared with vector controls are plotted. Two independent clones were selected in each strain, and the inductions were carried out in triplicates. Error bars represent the standard derivations. Full size image The off-target effects of ASRE(LacZ) were further determined by measuring the RNA levels of four genes with quantitative reverse-transcriptase PCR (RT–PCR) in cells transformed with ASRE(LacZ) or empty vector ( Fig. 3c ). The first two genes— eutE (accession number ECBD_1235) and yjcS (accession number ECBD_3947)—contain a single copy of the target sequence, whereas the ftsX gene (accession number ECBD_0279 ) contains a site with a single mismatch from the target ( Fig. 3c ), and the adhP (accession number ECBD_2161) gene does not harbour a similar site. A significant decrease in RNA level was observed only for lacZ but not for eutE or yjcS (both containing a single target site) or other RNAs ( Fig. 3c ). A possible reason may be that the LacZ RNA is induced together with ASRE expression, whereas other RNAs were occupied and protected by ribosomes before ASRE expression (see Discussion ). We developed a web-based application to help select the target sites of ASREs with minimal off-target effect ( http://www.unc.edu/usr-bin/ytsai/Puf.cgi ). This programme scans for all the 8-nt sequences in the target RNA and control RNAs for enriched 8-nt sequences. Multiple sequences or a long sequence (for example, a small genome) can be used as controls. The programme reports the 8-nt found only in the target sequence but not in the controls (the optimal 8-nt sites were ranked in the order of copy numbers). The possible secondary structure around the 8-nt binding site was also reported to ensure that there is no stably paired structure to prevent PUF binding (the maximal number of base pairs allowed is set as three). We empirically require at least three bases in the 8-nt binding sites to be unpaired. Gene silencing by ASRE in mitochondria To expand the application of ASREs as a gene-silencing tool, we generated a new ASRE to target mitochondria-encoded genes. Human mitochondria contain a circular DNA genome that encodes 13 proteins in the respiratory chain and mitochondrial transfer RNAs and ribosomal RNAs ( Fig. 4a ). Mutations in mitochondrial DNA are closely associated with various human diseases and ageing [15] , [16] ; however, it is difficult to study the functions of mitochondria-encoded genes because there are limited tools available to manipulate their expression. We engineered mitochondrial ASRE (mitoASRE) by including an N-terminal targeting peptide from ornithine transcarbamylase to facilitate mitochondrial protein import [17] ( Fig. 4a ). Control ASREs with inactive PIN or lacking mitochondrial targeting peptides were also generated ( Fig. 4b ). To minimize non-specific cleavage, we targeted a unique 8-nt (position 13,354 of NC_012920) in the mitochondrial genome within the NADH dehydrogenase subunit 5 (mtND5). Upon transient transfection into cultured cells, the mitoASREs were imported into mitochondria as judged by immunofluorescence staining ( Fig. 4c and Supplementary Fig. S8 ), whereas the control ASRE(ND5) was mainly found in the cytoplasm. We observed a small decrease (20–30%) of mtND5 mRNA in mitoASRE(ND5)-transfected cells using real-time RT–PCR, likely due to low transfection efficiency and/or inadequate protein production/import. 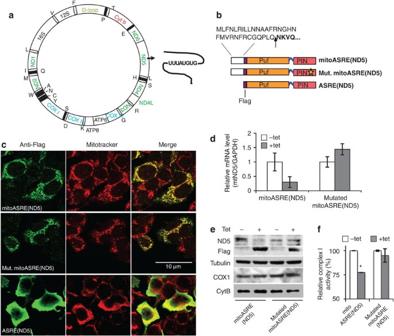Figure 4: Using ASRE to silence a mitochondrial gene. (a) A diagram of mitochondrial genome. The circular DNA genome of human mitochondrion contains genes coding for 13 proteins (colour coded for different oxidative phosphorylation complexes), two rRNA (16S and 12S) and 22 tRNAs. A unique sequence (TTTATGTG) in mtND5 coding region was chosen as the ASRE target. (b) Diagram of mitoASREs containing an N-terminal mitochondrial targeting peptide that, after translocation, will be cleaved (shown by an arrow). (c) Immunofluorescence of 293 cells expressing mitoASREs and a control ASRE. The mitochondria were stained with MitoTracker. (d) The changes of mtND5 RNA level 24 h after the tetracycline induction. Two independent inductions were carried out, and the real-time RT–PCR experiments were conducted in triplicates with glyceraldehyde 3-phosphate dehydrogenase as internal controls. The average of the relative mtND5 RNA levels compared with uninduced samples were plotted, with error bars indicating standard derivations. (e) Changes of mtND5 protein after induction. The levels of both mitochondrial encoded proteins (COX1 and cytB) and the nuclear encoded protein (tubulin) were measured as controls. (f) Changes of the complex I activity upon induction as measured with a spectrophotometric assay25. For each cell line, the activities relative to uninduced sample were plotted. Three independent inductions and mitochondrial preparations were conducted, and each sample was measured in triplicates. The mean and s.e. of all samples were plotted (*P=0.0014, paired Student'st-test). Figure 4: Using ASRE to silence a mitochondrial gene. ( a ) A diagram of mitochondrial genome. The circular DNA genome of human mitochondrion contains genes coding for 13 proteins (colour coded for different oxidative phosphorylation complexes), two rRNA (16S and 12S) and 22 tRNAs. A unique sequence (TTTATGTG) in mtND5 coding region was chosen as the ASRE target. ( b ) Diagram of mitoASREs containing an N-terminal mitochondrial targeting peptide that, after translocation, will be cleaved (shown by an arrow). ( c ) Immunofluorescence of 293 cells expressing mitoASREs and a control ASRE. The mitochondria were stained with MitoTracker. ( d ) The changes of mtND5 RNA level 24 h after the tetracycline induction. Two independent inductions were carried out, and the real-time RT–PCR experiments were conducted in triplicates with glyceraldehyde 3-phosphate dehydrogenase as internal controls. The average of the relative mtND5 RNA levels compared with uninduced samples were plotted, with error bars indicating standard derivations. ( e ) Changes of mtND5 protein after induction. The levels of both mitochondrial encoded proteins (COX1 and cytB) and the nuclear encoded protein (tubulin) were measured as controls. ( f ) Changes of the complex I activity upon induction as measured with a spectrophotometric assay [25] . For each cell line, the activities relative to uninduced sample were plotted. Three independent inductions and mitochondrial preparations were conducted, and each sample was measured in triplicates. The mean and s.e. of all samples were plotted (* P =0.0014, paired Student's t -test). Full size image For a more robust expression, we used the Flp-In T-REx system to generate stable cell lines that produce mitoASREs upon tetracycline induction. We observed an approximately 70% decrease of mtND5 RNA in cells expressing mitoASRE(ND5) compared with uninduced cells ( Fig. 4d ). Interestingly, cells expressing inactive mitoASRE increased the mtND5 RNA level compared with the uninduced cells. This unexpected result was reproduced in multiple inductions, possibly because the binding of inactive mitoASRE(ND5) stabilized mtND5 RNA. The mitoASRE(ND5), but not the inactive control, reduced ND5 protein level as judged by western blot ( Fig. 4e ). As controls, the levels of two additional mitochondrial proteins (COX1 and CytB) were found unchanged ( Fig. 4e ). We further measured the biosynthesis of all mitochondria-encoded proteins using a translation assay with S 35 -labelled methionine and emetine, and found that the biosynthesis of ND5, but not other mitochondria-encoded proteins, were significantly decreased by mitoASRE(ND5; Supplementary Fig. S9 ). As a control, the expression of mutated mitoASRE(ND5) did not affect mitochondrial protein synthesis, suggesting that the reduced level of ND5 translation is due to specific mRNA degradation. In addition, the off-target effects of mitoASRE(ND5) were evaluated by measuring the change in RNA levels for all mitochondrial protein-coding genes and rRNAs after tetracycline induction. We found that only the ND5 RNA showed a significant decrease (by 72%), whereas the levels of other RNAs did not change or slightly increased ( Supplementary Fig. S10a ). The cells expressing mitoASRE(ND5) showed a slow growth during the first 2–3 days of induction ( Supplementary Fig. S10b ); however, this phenotype is transient and the cells eventually recovered to normal growth. As mtND5 is a subunit of the mitochondrial respiratory complex I, we measured complex I activities after the induction of wt or mutated mitoASRE(ND5; Fig. 4f ). The mitoASRE(ND5), but not the inactive mutant, caused a modest but reproducible decrease in total complex I activity ( Fig. 4f , P =0.0014), consistent with previous clinical findings [18] , [19] . The detailed mechanism of how mtND5 silencing can affect cell metabolism is interesting but beyond the scope of this study. In this study, we engineered a series of RNA 'restriction enzymes' using rational protein design from different functional modules. Similar designs have been applied to artificial DNA enzymes (aka zinc-finger nucleases), where a zinc finger DNA-binding domain and a DNA-cleavage domain are combined [20] to target unique sequences within complex genomes [21] . However, restriction enzymes targeting RNA have not been discovered in nature and the creation of artificial enzymes resembling zinc-finger nucleases has been proven difficult, primarily because of limited understandings of a recognition code for RNA–protein interactions [22] . We have taken advantage of the specific RNA binding 'code' of the PUF domain and the endonuclease activity of the PIN domain. Generating this novel class of enzymes enables efficient and specific cleavage of diverse RNA targets both in vitro and in vivo . Key considerations for the successful generation of ASREs include selections of a sequence-specific RNA-binding domain, a suitable endonuclease domain, an optimal linker and a correct orientation of these elements. Our data suggest that the unique RNA recognition mode of the PUF domain renders ASREs the ability to specifically recognize a diverse panel of RNA targets without detectable cross activity between non-cognate ASRE/RNA pairs. We also demonstrate that the PIN domain of human SMG6 cleaves RNAs at specific sites only when fused to the C terminus of the PUF domain, but not in a reverse orientation ( Fig. 1b ). One possible explanation is that the PIN in PUF–PIN orientation can 'fold back' so that the active site faces the RNA bound by the PUF domain to specifically cleave the substrate ( Supplementary Fig. S11a ), whereas in the PIN–PUF orientation the PIN-active site faces away from PUF to cleave any nearby RNA ( Supplementary Fig. S11b ). Alternatively, the bridge region joined by the linker and the C-terminal residues of PIN could be very flexible, allowing non-specific RNA sequences to become accessible to the PIN-active site when ASRE is constructed in a PIN–PUF orientation ( Supplementary Fig. S11c ). We further found that medium-sized linkers (7–12 amino acids) rich in slightly polar hydrophilic amino acids are best suited for the design. When assuming the inter-domain linker in ASRE to adopt a structure similar to that in their native contexts, we found that linkers with α-helical or helix-coil-helix structures produced the most active ASREs, whereas linkers with 3 10 helix structures reduced the activity of ASREs ( Fig. 2 ). Furthermore, the linker length also affects the specificity of the enzyme: non-specific cleavage became apparent with linkers approaching ~20 Å in length ( Fig. 2 ), probably due to excess flexibility that allowed the PIN endonuclease domain to recognize and cleave any RNA. Alternatively, longer linkers might directly affect binding of PUF to the RNA (for example, by steric hindrance at RNA–PUF binding surfaces), leading to non-specific binding and cleavage by ASRE. Thus, the independent domain movement should be considered an important parameter in controlling non-specific cleavage. Several lines of evidence confirm that RNA cleavage by ASREs is indeed catalysed by the PIN domain of SMG6 as follows: (1) ASRE has the same cation preference as that of PIN ( Fig. 1e ), both requiring Mn 2+ for maximum activity [11] ; (2) a mutation in the active site of the PIN domain abolished ASRE activity; (3) non-specific RNA cleavage was observed when the PIN domain had too much flexibility to recognize any RNA (either with a long linker or a reverse PIN–PUF orientation), consistent with non-specific activities of the PIN domain [11] . The specificity of ASRE is determined by an 8-nt recognition site, which is similar to the length of the seed match for RNAi [23] . To minimize off-target effects during in vivo application, one might preferably select PUFs to recognize an 8-nt sequence present in multiple copies in the target RNA. Many factors might influence the ASRE efficiency. RNA structures may affect the specific recognition between PUF and target RNA, or change the accessibility of the PIN domain to the cleavage site, suggesting that when requiring efficient cleavage we should select target sites in regions that lack a stable structure. For in vivo applications, the expression window of ASRE may also affect its efficiency. For example, the expression of both T7-driven ASRE and chromosomal lacZ in E. coli were induced simultaneously with IPTG. As the T7 RNA polymerase is almost eight times faster than the bacterial RNA polymerase [24] , ASRE was presumably synthesized faster than lacZ , providing a time window for the ASRE to cleave lacZ mRNA. The observation that ASRE(lacZ) could specifically silence lacZ expression suggested that the ASRE can recognize its target with sufficiently high efficiency and affinity to overcome the protective effect of ribosomes. As an added benefit, the co-transcriptional binding of mRNA by ribosomes may limit low-affinity off-target effects of ASREs, as only the specific ASRE with high binding affinity could compete efficiently with ribosomes. One may also express ASRE from constitutive promoters to ensure that the ASRE is present when the target RNA is being synthesized. As the first generation of ASRE, there are various ways to optimize its activity and expand its application. For example, it may be possible to create ASREs that recognize a target of different length (other than 8-nt). ASREs capable of recognizing longer sites may minimize off-target effects, whereas a shorter targeting site will be helpful for probing RNA structures. In addition, the catalytic activity of ASRE may also be improved by using RNA endonuclease domains other than PIN, or by optimizing the PIN domain active site. Finally, the relative positions of the cleavage sites are probably affected by the conformation of the linker region, thus testing peptide linkers with different sequences, and structures will likely reduce the 'star activity' of ASREs so that the cleavage occurs at a single, predictable site. The modular design combining an RNA recognition domain with a functional domain has been applied in engineering artificial factors to modulate splicing [25] or to visualize RNAs in live cells [26] , and similar configurations may be applied to devise new proteins for specific manipulations of RNA. Construction and expression of ASREs The PUF domain of human Pum1 (residue 828–1,176) and the PIN domain of human Smg6 (residue 1,238–1,421) were amplified with PCR and joined by sequences encoding different peptide linkers designed according to amino acid propensity of known protein linkers ( http://www.ibi.vu.nl/programs/linkerdbwww ). The resulting fusion proteins were cloned in expression vector pT7HTb or pET43.1b, and purified for analyses of their activities. See Supplementary Methods for more details. Nomenclature of ASRE The ASREs were named according to the identity of their PUF domains, as most ASRE had the same PIN domain. Each PUF domain recognizes its 8-nt target sequence in an anti-parallel fashion, with the first repeat recognizing the eighth base and so on; wt PUF repeat: C terminus-R8R7R6R5R4R3R2R1-N terminus, RNA target: 5′-UGUAUAUA-3′. We named the targets of a modified PUF in a reverse order (from C to N terminus) with the number of mutated PUF repeat and the base recognized by the corresponding repeat. For example, RNA target 7u6g represents the 5′-UugAUAUA-3′ sequence, with the mutated base shown in lower case. The PUF domains were named by the mutated repeats and the number of mutated amino acid in each in each repeat is marked. For example, ASRE(6-2/7-2) has two mutated amino acids in each of sixth and seventh repeat, causing it to recognize the 7u6g RNA. See Supplementary Table S2 for more examples. Determination of the RNA cleavage site To determine the cleavage sites of ASREs, we extracted the 5′-and 3′-digestion products from denaturing urea–PAGE gels and used RACE to map both ends of the cleavage products. To map the 3′-end of the 5′-fragment, we used polyA polymerase to add a 10- to 30-nt poly-A tail at the end of 5′-fragment and reverse transcribed the resulting RNA with a poly-T-containing primer. The resulting complementary DNA was amplified by nested PCR, cloned in pcDNA3 and sequenced ( Supplementary Fig. S5a , left panel). To map the 5′-end of the 3′-cleavage product ( Supplementary Fig. S5a , right panel), the gel-extracted RNA was first reverse transcribed with a specific primer. The resulting cDNA was purified and elongated with terminal transferase in the presence of dATP. Second, strand synthesis was carried out using a poly-T-containing primer and Klenow fragment. The resulting product was PCR amplified, cloned and sequenced. Gene silencing by ASRE in bacterial cells E. coli BL21(DE3) was transformed with either empty vector pET43.1b, or the vector encoding ASRE(LacZ) or a control ASREs not targeting lacZ mRNA. Multiple colonies were selected in each sample to circumvent clonal variation. Protein expression of each clone was induced with 0.3 mM IPTG for 6 h at 37 °C. To measure β-galactosidase activity, cells were lysed with two rounds of sonication in cold buffer and the standard β-galactosidase activity assay for all lysates was carried out in a 96-well plate format as described previously [27] . Total protein concentrations of each sample were measured using the Bradford method to ensure equal amounts of total protein were used in the activity assays. To measure mRNA levels, total cellular RNA was purified with a Qiagen RNeasy kit and treated with DNase I. Equal amounts of total RNA (300–500 ng) from each sample were used to make first-strand cDNA by random priming (High-capacity cDNA reverse transcription kit from Applied Biosystem), and the lacZ mRNA were measured with quantitative PCR using SYBR green kit of Applied Biosystem. Immunoblotting with a monoclonal β-galactosidase antibody (Santa Cruz; catalogue number sc-56394) was used to measure β-galactosidase protein levels. Gene silencing in mitochondria A DNA fragment encoding the mitochondrial targeting signal from the ornithine transcarbamylase leader peptide followed by the Flag tag was synthesized and cloned into the expression vector pT7HTb at the 5′-end of ASRE. Additional mutations were introduced in the PUF domain of mitoASRE to make it recognize the 5′-UUAUGUG-3′ target. The resulting mitoASRE(ND5) were cloned into pcDNA3 vector, and then transfected into HeLa or 293T cells. The total RNAs and proteins were collected 24 h post transfection for real-time RT–PCR, immunofluorescence staining and western blots. To generate stable cell lines expressing mitoASRE, we subcloned mitoASRE(ND5) and controls into pcDNA5/FRT/TO vector and co-transfected these constructs with pOG44 plasmid into the Flp-In T-REx 293 cells (Invitrogen). Stably integrated cells were selected and induced as described in Supplementary Methods . Mitochondrial translation assay In vivo mitochondrial translation was conducted as previously described [28] , [29] . Briefly, cells harbouring mitoASRE(ND5) or mutated mitoASRE(ND5) expression vectors were induced with tetracycline for 24 h as described earlier and washed twice with DMEM media lacking cysteine and methionine, but supplemented with 10% dialysed FBS (purchased from Invitrogen). The cells were further cultured in this media for 2 h, treated with emetine for 10 min at a final concentration of 200 μg ml −1 to block cytoplasmic translation, and then incubated with the L-[S 35 ] methionine (150 μCi ml −1 ; Perkin Elmer) for 1 h. The total proteins of each sample were separated with 15% SDS–PAGE gels, and the dried gels were exposed to storage phosphor screen for 7 days at −80 °C and imaged on a Typhoon Trio + Scanner (GE Health Care). Activity assay for mitochondrial complex I The activity of mitochondrial complex I was measured using a spectrophotometric assay [30] . Briefly, the cells stably transfected with mitoASRE(ND5) or catalytically inactive mitoASRE(ND5) mutant were induced by 10 μg ml −1 tetracycline, and the mitochondria were purified by two centrifugation steps [30] . The protein contents of mitochondria preparation were quantified with Bradford method, and the mitochondria of 1 μg protein equivalent was incubated in 25 mM KPO4 buffer (pH 7.8) containing 3.5 mg ml −1 BSA, 60 μM dichlorophenol indophenol, 70 μM decylubiquinone, 1.0 μM antimycin-A and 0.2 mM NADH at 37 °C (ref. 30 ). Reduction of dichlorophenol indophenol was followed at OD 600 in the interval for 4 min. Difference in OD 600 was measured in triplicates and normalized against total mitochondrial protein. For each sample, we carried out three independent inductions and mitochondria preparations, the activity assays were performed in triplicates, and the mean activities relative to the uninduced samples were plotted ( Fig. 4f ). Paired t -test was performed using GraphPad Prism software. How to cite this article: Choudhury, R. et al . Engineering RNA endonucleases with customized sequence specificities. Nat. Commun. 3:1147 doi: 10.1038/ncomms2154 (2012).